Non-muscle myosin II regulates survival threshold of pluripotent stem cells Human pluripotent stem (hPS) cells such as human embryonic stem (hES) and induced pluripotent stem (hiPS) cells are vulnerable under single cell conditions, which hampers practical applications; yet, the mechanisms underlying this cell death remain elusive. In this paper, we demonstrate that treatment with a specific inhibitor of non-muscle myosin II (NMII), blebbistatin, enhances the survival of hPS cells under clonal density and suspension conditions, and, in combination with a synthetic matrix, supports a fully defined environment for self-renewal. Consistent with this, genetically engineered mouse embryonic stem cells lacking an isoform of NMII heavy chain (NMHCII), or hES cells expressing a short hairpin RNA to knock down NMHCII, show greater viability than controls. Moreover, NMII inhibition increases the expression of self-renewal regulators Oct3/4 and Nanog, suggesting a mechanistic connection between NMII and self-renewal. These results underscore the importance of the molecular motor, NMII, as a novel target for chemically engineering the survival and self-renewal of hPS cells. Human pluripotent stem (hPS) cells including human embryonic stem (hES) and induced pluripotent stem (hiPS) cells are able to replicate themselves (self-renew) while retaining their ability to give rise to any type of specialized cells in the adult body (pluripotency). hPS cells are therefore promising sources for large-scale drug screenings or future cell-based therapeutics to treat diseases such as diabetes mellitus and spinal cord injuries [1] , [2] , [3] , [4] , [5] . Despite their potential clinical and industrial demand, the technical advance to control hPS cell growth remains hindered mainly because of underdeveloped culture methods and their low viability in clonal density or suspension conditions, which limits genetic manipulation and differentiation procedures [6] , [7] . Neurotrophins have been reported to protect hES cells from cell death through activation of Trk receptors [8] . More recently, a study showed a robust increase in hES cell survival by treatment with Y-27632, a chemical inhibitor of Rho-associated kinase (ROCK), at a level exceeding that of neurotrophins or other apoptosis inhibitors, although underlying mechanisms remained unclear [9] . There are multiple substrates regulated by ROCK [10] . In addition, Y-27632 affects several kinases other than ROCK, such as PRK2 and citron kinase [10] . The culture environment of hPS cells comprises two major elements, culture medium and extracellular matrix (ECM) coating, the latter of which include Matrigel, a cocktail of mouse tumour-derived ECM widely used for the feeder-free culture method [11] , [12] . Compared with the rapid progress in basic studies on self-renewal, less practical advances have been made in the methods to support self-renewal of hPS cells. Although fully defined culture medium is now available [13] , [14] , because of the complexity of the structural components of ECM and insufficient accumulation of basic studies on cellular interactions of hPS cells, the development of fully characterized and simplified coating methods still remains a major challenge [12] . We have previously demonstrated that non-muscle myosin II (NMII), a two-headed conventional myosin, has an essential role in the regulation of cellular interactions of hES cells, and NMII has been placed downstream of Rho-Rock signalling [15] . NMII has key roles in the broad ranges of basic biological functions, such as mitosis, migration and polarization conserved from unicellular organisms to humans [16] , [17] . Several studies also indicated the involvement of NMII in apoptotic processes in mammalian cells such as neural cells and fibroblasts [18] , [19] . To understand mechanisms underlying cell death in hPS cells and to find a new molecular target to engineer the survival threshold and cell growth under defined environments, we sought to determine the role of NMII for cell viability and self-renewal. We have found that pharmacological or genetic inhibition of NMII is sufficient to enhance survival of hPS cells under single cell growth conditions, and is able to increase expression levels of self-renewal regulators such as Oct3/4 and Nanog. Furthermore, with a pharmacological inhibitor of NMII, blebbistatin, we have developed novel fully defined and simplified culture conditions for self-renewal of hPS cells. NMII inhibition by blebbistatin enhances cloning efficiency NMII heavy chain (NMHCII) has three isoforms [16] , of which NMHCIIA and NMHCIIB but not NMHCIIC are readily detectable in hES cells by immunoblot analysis ( Fig. 1a ). Immunocytochemical analysis demonstrated that both isoforms were predominantly localized to plasma membranes in the undifferentiated hPS cells, consistent with their role in cell–cell contacts ( Fig. 1a ). To evaluate the function of NMII in cell death of hPS cells, we used blebbistatin, a synthetic chemical compound that effectively and reversibly blocks the ATPase activity of NMII, thereby suppressing motor function [20] . We first tested the viability of hES and hiPS cells plated on Matrigel-coated plates in mTeSR at clonal density, which is an initial critical hurdle in the establishment of individual clonal lines. Single hiPS cells were plated in each well of Matrigel-coated 96-well plates and undifferentiated colony formation was evaluated by alkaline phosphatase (ALP) staining, as well as by immunocytochemistry, using an antibody against a pluripotency marker, Oct3/4, at 7 days after plating. Although no or only a few colonies were formed under the control condition at 7 days after plating, approximately 30% of wells contained single colonies when cells were treated with blebbistatin (0.47±0.25% for control versus 29±4.3% with blebbistatin, P <0.01) ( Fig. 1b,c ). Some of the colonies were selected, further expanded and determined to be pluripotent through a series of molecular and functional analyses, including detection of pluripotency markers and in vivo differentiation assays ( Supplementary Fig. S1a–c ). This cloning efficiency was comparable to that using Y-27632 (22±7.5%) ( Fig. 1c and Supplementary Fig. S1d ) as reported previously [9] . 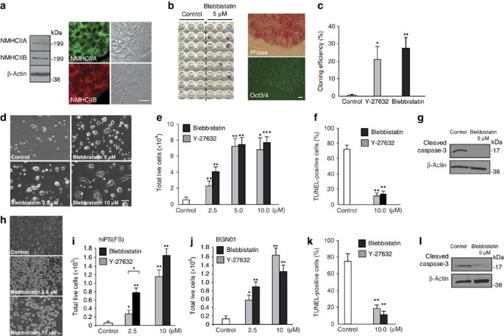Figure 1: Inhibition of NMII by blebbistatin enhances survival of hPS cells under clonal and suspension culture conditions. (a) Expression of NMHCIIA and IIB in hES cells as determined by immunoblot and immunocytochemical analyses. (b) Clonal assay of hiPS cells evaluated by alkaline phosphatase (ALP) assay (left panel) and immunocytochemistry using Oct3/4 antibody (right panel). hiPS cells were plated in the presence or absence of blebbistatin or Y-27632. (c) Cloning efficiency was determined by the ratio of the number of wells with an ALP-positive colony to the number of wells seeded. (d–g) Cell viability assay of hiPS cells under adherence conditions (seeMethodssection). Cells were photographed after 24 h in culture (d) and the number of viable cells was counted by Trypan blue exclusion assay (e). The same experiment was repeated at least three times per cell line, and representative data are shown. (f) Evaluation of apoptosis of hiPS cells. Cells used for cell viability assay in (e) were subjected to TUNEL assay. (g) Cells plated under the same condition as shown in (e) were evaluated by immunoblot analysis using an antibody against cleaved caspase-3. (h–l) Blebbistatin treatment increases survival of hPS cells in suspension culture. hiPS(FS) or hES (BGN01) cells were grown in suspension culture in hESm in the presence or absence of blebbistatin or Y-27632 for 2 days, subsequently photographed (hiPS cells are shown) (h), and subjected to live cell counting for hiPS (i) and hES (j) cells. TUNEL assay (k) and immunoblot analysis detecting cleaved caspase-3 (l) were also carried out (data from hiPS cells are shown). For immunoblot analysis, β-actin was used as a loading control. Data are mean±s.d., *P<0.05, **P<0.01, ***P<0.001,n=3. Scale bars, 25 μm. Figure 1: Inhibition of NMII by blebbistatin enhances survival of hPS cells under clonal and suspension culture conditions. ( a ) Expression of NMHCIIA and IIB in hES cells as determined by immunoblot and immunocytochemical analyses. ( b ) Clonal assay of hiPS cells evaluated by alkaline phosphatase (ALP) assay (left panel) and immunocytochemistry using Oct3/4 antibody (right panel). hiPS cells were plated in the presence or absence of blebbistatin or Y-27632. ( c ) Cloning efficiency was determined by the ratio of the number of wells with an ALP-positive colony to the number of wells seeded. ( d – g ) Cell viability assay of hiPS cells under adherence conditions (see Methods section). Cells were photographed after 24 h in culture ( d ) and the number of viable cells was counted by Trypan blue exclusion assay ( e ). The same experiment was repeated at least three times per cell line, and representative data are shown. ( f ) Evaluation of apoptosis of hiPS cells. Cells used for cell viability assay in ( e ) were subjected to TUNEL assay. ( g ) Cells plated under the same condition as shown in ( e ) were evaluated by immunoblot analysis using an antibody against cleaved caspase-3. ( h – l ) Blebbistatin treatment increases survival of hPS cells in suspension culture. hiPS(FS) or hES (BGN01) cells were grown in suspension culture in hESm in the presence or absence of blebbistatin or Y-27632 for 2 days, subsequently photographed (hiPS cells are shown) ( h ), and subjected to live cell counting for hiPS ( i ) and hES ( j ) cells. TUNEL assay ( k ) and immunoblot analysis detecting cleaved caspase-3 ( l ) were also carried out (data from hiPS cells are shown). For immunoblot analysis, β-actin was used as a loading control. Data are mean±s.d., * P <0.05, ** P <0.01, *** P <0.001, n =3. Scale bars, 25 μm. Full size image Increased survival in adhesive conditions by blebbistatin Next, we evaluated whether the cytoprotective effect of blebbistatin was detectable within a short period of time after plating. For all of the hPS cell culture experiments, cells were collected by trypsinization, and extensively triturated by rigorous pipetting to obtain single cells to be plated. Cells (1×10 5 cells per well, 12-well plates) grown in mTeSR were treated with or without blebbistatin at different concentrations, and viability was evaluated by direct cell counting at 24 h after plating. hiPS cells treated with blebbistatin survived in significantly higher numbers than did control cells (the highest effect was observed between 5 and 10 μM) when cultured on different substrates such as poly- D -lysine (PDL) (7.9±0.6×10 4 cells at 10 μM blebbistatin versus 0.5±0.26×10 4 cells for control, n =3, P <0.001) and Matrigel coating (8.6±0.6×10 4 cells at 10 μM blebbistatin versus 1.8±0.25×10 4 cells for control, n =3, P <0.01) ( Fig. 1d,e , and Supplementary Fig. S1e–g ). We also tested Y-27632 under the same conditions side by side, and found that the survival effect of blebbistatin was comparable to that of Y-27632 (7.2±1.1×10 4 cells at 10 μM on PDL, n =3, P <0.05) ( Fig. 1d,e and Supplementary Fig. S1e ). This result inversely correlated with the level of apoptosis detected by terminal deoxynucleotidyltransferase dUTP nick end labelling (TUNEL) assay. More than 70% of cells in the control condition were positive for TUNEL staining, whereas cells treated with blebbistatin exhibited significantly lower numbers of TUNEL-positive cells (73±2.5% for control versus 11±3.8% with blebbistatin, n =3, P <0.01) ( Fig. 1f ). This result was further confirmed by another indicator of apopotosis, cleaved caspase-3, which, by immunoblot analysis, was undetectable in blebbistatin-treated cells, indicating a reduced number of apoptotic cells after blebbistatin treatment ( Fig. 1g ). Inhibition of NMII prevents cell death in suspension culture To test whether blebbistatin is also effective on cells without cell–matrix adhesion, cells were grown in suspension culture, which is a common primary step for the generation of embryoid bodies in standard differentiation protocols. Cells were trypsinized and rigorously triturated to single cells and plated in non-conditioned human ES medium (hESm) with or without blebbistatin for 48 h. Remarkably, blebbistatin treatment increased the viability of hiPS cells to a level significantly higher than that of controls under suspension conditions (1.6±0.12×10 5 cells at 10 μM blebbistatin versus 0.05±0.02×10 5 cells, n =3, P <0.01) ( Fig. 1h,i ). hES cells and the other independent hiPS cell lines showed a comparable survival effect by blebbistatin ( Fig. 1j and Supplementary Fig. S2a ). This result was supported by TUNEL and cleaved caspase-3 assays demonstrating significantly lower levels of apoptosis in the blebbistatin treatment condition ( Fig. 1k,l and Supplementary Fig. S2b ). It is of note, however, that at a lower concentration, blebbistatin treatment consistently yielded higher viability than Y-27632, whereas at 10 μM, the survival effect of blebbistatin or Y-27632 was variable depending on individual cell lines ( Fig. 1i,j and Supplementary Fig. S2a ). Thus, blebbistatin provides an alternative strategy to protect hPS cells according to dosage and effectiveness on individual cell lines. To evaluate whether the observed effect of blebbistatin was due to the specific activity of the compound, we tested two available enantiomers of blebbistatin. As expected, an inactive form of blebbistatin, blebbistatin (+), did not show any significant effect on cell survival at 24 h after treatment, whereas an active enantiomer, blebbistatin (−), demonstrated an effect comparable to that of the racemic mixture, blebbistatin (±), which we mainly used in the study ( Fig. 2a ). Interestingly, ML-7, an inhibitor of myosin light chain kinase, which is involved in the regulation of myosin-mediated contractility and apoptosis in other cell types [18] , [19] , did not show a significant effect on survival ( Fig. 2b and Supplementary Fig. S1h ). This suggests that the function of NMII in the cell death regulation of pluripotent stem cells may be mainly controlled by ROCK through myosin light chain phosphatase [10] rather than myosin light chain kinase. Consistent with this possibility, combined treatment with blebbistatin and Y-27632 at different concentrations for 24 h did not show substantial additive or synergistic effects on survival of hPS cells ( Fig. 2c ). 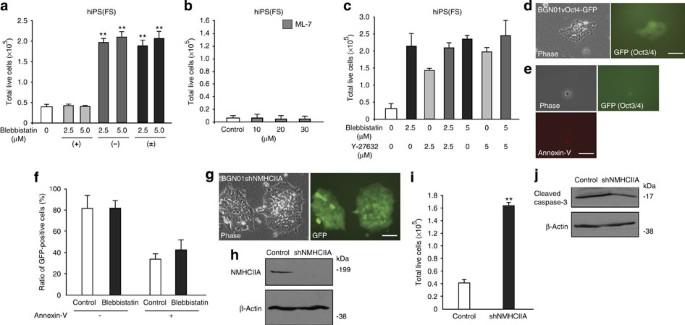Figure 2: Effect of blebbistatin enantiomers or shRNA-mediated knockdown of NMHCIIA on cell death of hPS cells grown under suspension conditions. (a) hiPS cells were grown in suspension culture conditions in the presence of the plus or minus enantiomer of blebbistatin at different concentrations in hESm for 24 h, and subjected to live cell counting. (b) hiPS cells grown under suspension condition in hESm were treated with ML-7 at various concentrations for 2 days. (c) hiPS cells were cultured under suspension conditions in hESm with combinations of blebbistatin and Y-27632 at different concentrations for 24 h, and subjected to live cell counting. (d–f) Annexin-V binding assay using the Oct3-GFP hES reporter line. BGN01vOct4-GFP reporter cells were grown in suspension conditions in the presence or absence of 5 μM blebbistatin in hESm for 24 h, and evaluated by annexin-V binding assay. (d) Morphology and GFP expression of hES reporter cells grown under feeder-free conditions. (e) Images of a representative single cell that is positive for both GFP and annexin-V. (f) Ratios of GFP-positive cells in annexin-V-positive or -negative cell populations under control or blebbistatin-treated conditions. (g) Morphology and GFP expression of BGN01 cells stably expressing NMHCIIA shRNA (shNMHCIIA). BGN01 cells were infected with a lentiviral vector carrying NMHCIIA shRNA sequences and GFP reporter. Individual lines were established and confirmed for knockdown of NMHCIIA by immunoblot analysis (h). (i,j) Knockdown of NMHCIIA by shRNA enhances survival of hES cells in the suspension culture. hES cells with stable knockdown of NMHCIIA were cultured under suspension conditions in hESm for 24 h, and subjected to live cell counting (i) and immunoblot analysis using cleaved caspase-3 antibody (j). β-Actin was used as a loading control. Data are mean±s.d., **P<0.01,n=3. Scale bars, 25 μm. Figure 2: Effect of blebbistatin enantiomers or shRNA-mediated knockdown of NMHCIIA on cell death of hPS cells grown under suspension conditions. ( a ) hiPS cells were grown in suspension culture conditions in the presence of the plus or minus enantiomer of blebbistatin at different concentrations in hESm for 24 h, and subjected to live cell counting. ( b ) hiPS cells grown under suspension condition in hESm were treated with ML-7 at various concentrations for 2 days. ( c ) hiPS cells were cultured under suspension conditions in hESm with combinations of blebbistatin and Y-27632 at different concentrations for 24 h, and subjected to live cell counting. ( d – f ) Annexin-V binding assay using the Oct3-GFP hES reporter line. BGN01vOct4-GFP reporter cells were grown in suspension conditions in the presence or absence of 5 μM blebbistatin in hESm for 24 h, and evaluated by annexin-V binding assay. ( d ) Morphology and GFP expression of hES reporter cells grown under feeder-free conditions. ( e ) Images of a representative single cell that is positive for both GFP and annexin-V. ( f ) Ratios of GFP-positive cells in annexin-V-positive or -negative cell populations under control or blebbistatin-treated conditions. ( g ) Morphology and GFP expression of BGN01 cells stably expressing NMHCIIA shRNA (shNMHCIIA). BGN01 cells were infected with a lentiviral vector carrying NMHCIIA shRNA sequences and GFP reporter. Individual lines were established and confirmed for knockdown of NMHCIIA by immunoblot analysis ( h ). ( i , j ) Knockdown of NMHCIIA by shRNA enhances survival of hES cells in the suspension culture. hES cells with stable knockdown of NMHCIIA were cultured under suspension conditions in hESm for 24 h, and subjected to live cell counting ( i ) and immunoblot analysis using cleaved caspase-3 antibody ( j ). β-Actin was used as a loading control. Data are mean±s.d., ** P <0.01, n =3. Scale bars, 25 μm. Full size image Several reports have indicated that hES cells show heterogeneous expression patterns of pluripotency markers such as Oct3/4 and Nanog, and exhibit distinct differentiation propensities [21] , [22] , [23] . To exclude the possibility that the cells responding to blebbistatin are biased to particular populations of hES cells such as differentiating cells, we took advantage of an hES cell reporter line, BGN01v Oct4-GFP, in which green fluorescent protein (GFP) is driven by the Oct3/4 promoter, allowing us to monitor the transcriptional activity of Oct3/4. More than 95% of reporter cells expressed GFP under the regular feeder-free culture condition, as determined by fluorescence microscopy ( Fig. 2d ). The reporter hES cells were cultured under suspension conditions for 24 h as described above, and subsequently evaluated by annexin-V staining to identify apoptotic cells ( Fig. 2e ). Cells treated with 5 μM blebbistatin demonstrated an increase in the percentage of annexin-V-negative cells (74±4% plus belbbistatin versus 38±8% in control, P <0.01), of which the percentage of GFP-positive cells was 80±7% ( Fig. 2f ). This suggests that the cell population that survived as a result of blebbistatin treatment was not biased to minor populations of hES cells such as differentiated cells, but rather represents the original cell population that consisted of mostly undifferentiated cells. In both control and blebbistatin-treated cells, many annexin-V-positive cells expressed no or relatively low levels of GFP as compared with annexin-negative cells, indicating that cells undergoing apoptosis may downregulate Oct3/4 transcriptional activity because of stress responses or other unknown mechanisms ( Fig. 2f ). Synthetic compounds could in general affect multiple substrates besides the main target. It is therefore still possible that the effect on cell survival by blebbistatin may be mediated by unknown functions affecting molecules other than NMII. To verify that the inhibition of NMII is sufficient to enhance survival of hPS cells, we used a lentiviral vector carrying short hairpin RNA (shRNA) to knock down NMHCIIA. BGN01 cells constitutively expressing shRNA led to stable knockdown of NMHCIIA, and demonstrated significantly higher viability than control cells under suspension culture conditions (1.62±0.06×10 5 cells plus shRNA versus 0.4±0.05×10 5 cells in controls, n =3, P <0.01), further confirming the essential role of NMII for survival of hPS cells ( Fig. 2g–j ). Enhanced survival of mES cells lacking NMHCIIA To test whether the observed role of NMII in cell viability of hPS cells is also conserved in mice, we used mutant mouse embryonic stem (mES) cells in which both alleles of the NMHCIIA gene are disrupted (NMHCIIA − /A − ) [24] ( Fig. 3a , full gels shown in Supplementary Fig. S3 ). The cell–cell contacts of mutant cells were severely impaired as previously reported [24] ( Fig. 3b ). NMHCIIA − /A − mES cells exhibited significantly higher viability than the parental line (RW4) at 24 h after plating (1.3±0.3×10 5 cells for NMHCIIA − /A − versus 0.4±0.1×10 5 cells for controls, n =3, P <0.05) ( Fig. 3c,d ), consistent with the data using blebbistatin for hPS cells. The level of apoptosis was also determined by TUNEL assay, demonstrating considerably lower numbers of TUNEL-positive mutant cells as compared with wild-type mES cells ( Fig. 3e ). 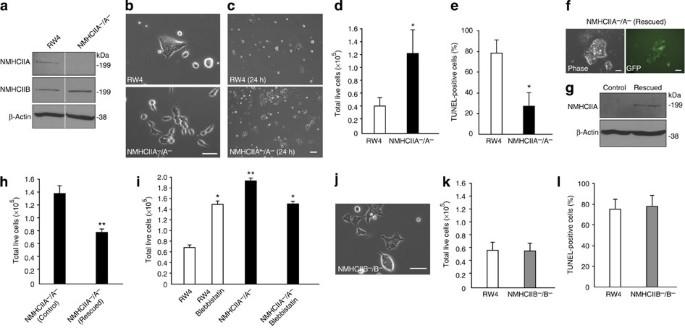Figure 3: Enhanced survival rate of NMHCIIA−/A−mES cells. (a) Expression of NMHCIIA and NMHCIIB in parental wild-type (RW4) and NMHCIIA−/A−mutant mES cells was evaluated by immunoblot analysis. (b) Morphology of RW4 and NMHCIIA−/A−mutant cells grown on gelatin-coated plates. The mutant cells show loose cell–cell contact, whereas RW4 cells exhibit tight cell–cell adhesions. (c–e) NMHCIIA−/A−mES cells survive at a higher rate than RW4. Cells were plated at 1×105cells per well on gelatin-coated 12-well plates in triplicate. After 24 h, cells were photographed (c), and evaluated by live cell counting (d) and by TUNEL assay (e). (f–h) Rescue of the phenotype of mutant mES cells. NMHCIIA−/A−mES cells were transfected with a plasmid construct carrying GFP-tagged NMHCIIA complementary DNA. The transfected cells were photographed (f), evaluated by immunoblot analysis using an antibody against NMHCIIA (g) and subjected to cell viability assay under suspension conditions (h). (i) Effect of blebbistatin on survival of mES cells. Wild-type (RW4) or NMHCIIA−/A−mES cells were grown in the suspension condition in the presence or absence of 5 μM blebbistatin for 24 h, and subjected to live cell counting. (j) Phase contrast image of NMHCIIB−/B−mES cells. Cells maintain cell–cell adhesions. (k,l) NMHCIIB−/B−mES cells were plated as described above and cell viability (k) and TUNEL (l) assays were carried out. β-Actin was used as a loading control. Data are mean±s.d., *P<0.05, **P<0.01,n=3. Scale bars, 25 μm. Figure 3: Enhanced survival rate of NMHCIIA − /A − mES cells. ( a ) Expression of NMHCIIA and NMHCIIB in parental wild-type (RW4) and NMHCIIA − /A − mutant mES cells was evaluated by immunoblot analysis. ( b ) Morphology of RW4 and NMHCIIA − /A − mutant cells grown on gelatin-coated plates. The mutant cells show loose cell–cell contact, whereas RW4 cells exhibit tight cell–cell adhesions. ( c – e ) NMHCIIA − /A − mES cells survive at a higher rate than RW4. Cells were plated at 1×10 5 cells per well on gelatin-coated 12-well plates in triplicate. After 24 h, cells were photographed ( c ), and evaluated by live cell counting ( d ) and by TUNEL assay ( e ). ( f – h ) Rescue of the phenotype of mutant mES cells. NMHCIIA − /A − mES cells were transfected with a plasmid construct carrying GFP-tagged NMHCIIA complementary DNA. The transfected cells were photographed ( f ), evaluated by immunoblot analysis using an antibody against NMHCIIA ( g ) and subjected to cell viability assay under suspension conditions ( h ). ( i ) Effect of blebbistatin on survival of mES cells. Wild-type (RW4) or NMHCIIA − /A − mES cells were grown in the suspension condition in the presence or absence of 5 μM blebbistatin for 24 h, and subjected to live cell counting. ( j ) Phase contrast image of NMHCIIB − /B − mES cells. Cells maintain cell–cell adhesions. ( k , l ) NMHCIIB − /B − mES cells were plated as described above and cell viability ( k ) and TUNEL ( l ) assays were carried out. β-Actin was used as a loading control. Data are mean±s.d., * P <0.05, ** P <0.01, n =3. Scale bars, 25 μm. Full size image To verify that the enhanced survival is due to the lack of NMHCIIA, we evaluated whether the observed phenotype can be rescued by reintroducing the NMHCIIA complementary DNA into the mutant ( Fig. 3f,g ). Mutant cells transfected with the GFP-tagged NMHCIIA complementary DNA exhibited reduced survival as compared with mutant cells transfected with a control GFP plasmid (0.78±0.05×10 5 cells plus NMHCIIA versus 1.38±0.12×10 5 cells transfected with a control plasmid, n =3, P <0.01), indicating that NMHCIIA is responsible for the altered survival of mES cells ( Fig. 3h ). We also found that blebbistatin effectively increased the viability of wild-type mES cells (1.48±0.07×10 5 cells plus blebbistatin versus 0.64±0.06×10 5 in control, n =3, P <0.05) as it did for hPS cells, whereas the compound treatment did not further enhance the survival of mutant mES cells lacking NMHCIIA ( Fig. 3i ). It has been suggested that the two isoforms of NMII, NMIIA and NMIIB, can have distinct functions in cell adhesion, migration and contractility [24] , [25] . We therefore evaluated whether NMIIB also has a role in the regulation of cell survival by using mutant mES cells genetically lacking NMHCIIB (NMHCIIB − /B − ) [26] ( Fig. 3j ). In contrast to the remarkable increase in the viability of NMHCIIA − /A − mES cells, the NMHCIIB mutant showed a survival rate similar to that of wild-type mES cells (0.54±0.1×10 5 cells versus 0.55±0.14×10 5 cells, n =3) ( Fig. 3k,l ). These results indicate that distinct regulatory mechanisms may control each isoform of NMII in the regulation of cell death of pluripotent stem cells, as is the case with cell adhesion and migration [24] , [25] , although other possibilities such as different amounts of each isoform in ES cells (81±7% NMHCIIA, 19±7% MHCIIB) need to be considered. Mechanistic link between NMII and self-renewal regulators We have previously identified a group of genes that were specifically enriched in the undifferentiated state of hES cells by conducting microarray analysis [27] . In searching the array database, we recognized that NMHCIIA transcripts were significantly enriched in the differentiated state of hES cells ( Supplementary Table S1 ), suggesting a potential molecular link between self-renewal/differentiation programs and NMII. We therefore decided to investigate whether self-renewal regulators such as Oct3/4 and Nanog [28] , [29] , [30] and NMII are mechanistically connected in hPS cells. hiPS or hES cells were grown in either mTeSR, which supports the undifferentiated state [13] , or non-conditioned hESm, which induces passive differentiation in the presence or absence of blebbistatin at different concentrations for 48 h [31] . hES cells treated with blebbistatin demonstrated elevated levels of both Oct3/4 and Nanog transcription factors in a dose-dependent manner under both medium conditions, as determined by quantitative reverse transcription–PCR and immunoblot analysis ( Fig. 4a–d , full gels for Fig. 4c are shown in Supplementary Fig. S4 ). Expression of the other pluripotency marker gene, Rex-1, and lack of expression of differentiation-related marker genes were confirmed by the conventional PCR ( Fig. 4e ). Immunocytochemical analysis showed higher expression levels of Oct3/4 in cells treated with blebbistatin under differentiation conditions ( Fig. 4f ). We also found that Y-27632 treatment of hES cells also showed a moderate increase in the expression of Oct3/4 by immunoblot analysis ( Supplementary Fig. S5 ). To determine whether this connection is also conserved in mice, we tested mES cells grown in the presence or absence of leukaemia inhibitory factor for 2 days. Consistent with the data from hES cells, both self-renewal regulators, Oct3/4 and Nanog, were expressed at substantially higher protein levels in NMHCIIA − /A − mES cells as compared with the parental cells under each condition ( Fig. 4g,h ). These data collectively suggest that NMII may function as a causal rather than as a consequential factor in the negative regulation of self-renewal in both human and mouse pluripotent stem cells. Although the underlying mechanisms are currently unknown, this connection could be mediated by the interactions between NMII and β1 integrin at focal adhesions which, in turn, activate multiple pathways, including ERK signalling, which has been implicated in differentiation of ES cells [32] , [33] . Alternatively, NMII may crosstalk with other self-renewal pathways such as transforming growth factor-β, PI3 kinase and Wnt signalling [30] , [34] through as yet unidentified molecular trafficking mechanisms. Nevertheless, the upregulation of self-renewal regulators by inhibition of NMII may contribute to the enhanced survival of self-renewing pluripotent stem cells. 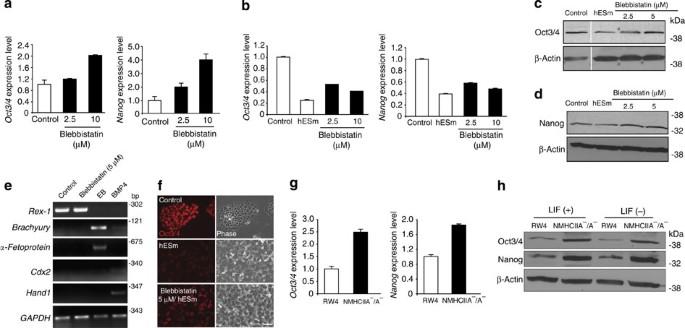Figure 4: Inhibition of NMII enhances expression of self-renewal regulators in human and mouse pluripotent stem cells. (a–d) hES cells were plated at 1×105cells per well on Matrigel-coated six-well plates in mTeSR without blebbistatin. After 24 h, the medium was changed to fresh mTeSR or hESm with or without blebbistatin at different concentrations. At 48 h after switching medium, cells were collected for RNA or protein extraction.Oct3/4andNanogexpression was determined by quantitative reverse transcription–PCR from cells grown in mTeSR (a) or hESm (b), or by immunoblot analysis from cells grown in hESm (c,d). The condition of cells grown in mTeSR without blebbistatin is indicated as 'control'. Expression levels on theyaxis are shown in arbitrary units (control is set to 1.0). (e) The same complementary DNA (cDNA) samples as used in (a–d) were subjected to conventional PCR using primers specific for a pluripotency marker,Rex-1, and differentiation-related markers such asbrachyury(mesoderm), α-fetoprotein(endoderm),Cdx2(trophectoderm) andHand1(trophectoderm).GAPDHwas used as a loading control. cDNA samples obtained from differentiated hES cells through embryoid body (EB) formation for 21 days or through BMP4 (100 ng ml−1) treatment for 5 days were used as differentiation controls. (f) Cells grown under the same conditions (hESm with or without 5 μM blebbistatin) were also subjected to immunocytochemistry to detect Oct3/4 expression. The images were captured with exactly the same parameters between each condition, including exposure time for each filter and magnifications. Phase contrast images showed that cells grown in hESm exhibited a large and flat morphology indicative of differentiation, whereas cells grown in mTeSR (control) maintained a compact and tight morphology. Scale bar, 25 μm. (g) Expression ofOct3/4andNanogin wild-type (RW4) and NMHCIIA−/A−mES cells grown in the presence of leukaemia inhibitory factor (LIF) was analysed by quantitative reverse transcription–PCR (QPCR). Control is set to 1.0. (h) The same set of mES cell lines grown in the presence or absence of LIF for 2 days was evaluated by immunoblot analysis. For QPCR, the data were normalized to the expression level of β-Actin. β-Actin was used as a loading control for immunoblot analyses. Data are mean±s.d.,n=3. Figure 4: Inhibition of NMII enhances expression of self-renewal regulators in human and mouse pluripotent stem cells. ( a – d ) hES cells were plated at 1×10 5 cells per well on Matrigel-coated six-well plates in mTeSR without blebbistatin. After 24 h, the medium was changed to fresh mTeSR or hESm with or without blebbistatin at different concentrations. At 48 h after switching medium, cells were collected for RNA or protein extraction. Oct3/4 and Nanog expression was determined by quantitative reverse transcription–PCR from cells grown in mTeSR ( a ) or hESm ( b ), or by immunoblot analysis from cells grown in hESm ( c , d ). The condition of cells grown in mTeSR without blebbistatin is indicated as 'control'. Expression levels on the y axis are shown in arbitrary units (control is set to 1.0). ( e ) The same complementary DNA (cDNA) samples as used in ( a – d ) were subjected to conventional PCR using primers specific for a pluripotency marker, Rex-1 , and differentiation-related markers such as brachyury (mesoderm), α -fetoprotein (endoderm), Cdx2 (trophectoderm) and Hand1 (trophectoderm). GAPDH was used as a loading control. cDNA samples obtained from differentiated hES cells through embryoid body (EB) formation for 21 days or through BMP4 (100 ng ml −1 ) treatment for 5 days were used as differentiation controls. ( f ) Cells grown under the same conditions (hESm with or without 5 μM blebbistatin) were also subjected to immunocytochemistry to detect Oct3/4 expression. The images were captured with exactly the same parameters between each condition, including exposure time for each filter and magnifications. Phase contrast images showed that cells grown in hESm exhibited a large and flat morphology indicative of differentiation, whereas cells grown in mTeSR (control) maintained a compact and tight morphology. Scale bar, 25 μm. ( g ) Expression of Oct3/4 and Nanog in wild-type (RW4) and NMHCIIA − /A − mES cells grown in the presence of leukaemia inhibitory factor (LIF) was analysed by quantitative reverse transcription–PCR (QPCR). Control is set to 1.0. ( h ) The same set of mES cell lines grown in the presence or absence of LIF for 2 days was evaluated by immunoblot analysis. For QPCR, the data were normalized to the expression level of β -Actin . β-Actin was used as a loading control for immunoblot analyses. Data are mean±s.d., n =3. Full size image Establishment of a fully defined condition for hPS cells We have recently reported that Y-27632 treatment enables hES cells to self-renew on PDL coating, a substrate on which hES cells do not normally grow [15] . Because PDL is a chemically synthesized substrate, unlike Matrigel, a mouse tumour-derived extract, we established a fully defined condition for self-renewal of hES cells using a defined medium, mTeSR [15] . As blebbistatin accurately replicates all of the effects of Y-27632 on both hES and iPS cells, we tested whether blebbistatin alone can fully replace Y-27632 in the defined culture condition. Blebbistatin was used at concentrations between 2.5 and 5 μM, which are the minimum concentrations sufficient for supporting self-renewal but not affecting cell–cell adhesions [15] . The maintenance of typical undifferentiated morphology and expression of pluripotency markers was confirmed in each line after 20 passages under this defined condition ( Fig. 5a–d ). hiPS or hES cells were able to self-renew on PDL at a constant growth rate comparable to that of cells treated with Y-27632 or cells grown under regular feeder-free conditions using Matrigel [11] ( Fig. 5e ). To assess full differentiation functions in vivo , the passaged cells were subjected to teratoma assay by subcutaneous injection into severe combined immunodeficient (SCID)/beige mice. The teratoma samples were examined by histological analysis and determined to contain differentiated tissues derived from all three germ layers, such as melanocytes (ectoderm), neuronal tissue (ectoderm), bone (mesoderm), skeletal muscle (mesoderm), gastrointestinal-like mucosal epithelium with goblet cells (endoderm) and glomeruli (endoderm) ( Fig. 5f ). This was further validated by immunohistochemistry detecting specialized cell-specific marker proteins ( Fig. 5g ). These results confirmed that hES or hiPS cells grown under the defined condition with blebbistatin can self-renew for an extended period of time without compromising multidifferentiation capacities, verifying the full reversibility of the effect of blebbistatin. The cells were determined to maintain genomic integrity as evaluated by karyotyping (hiPS cells in Fig. 5h , and hES cells in Supplementary Fig. S6 ). It has been reported that the strong inhibition of NMII by blebbistatin at high concentrations (50–100 μM) affects cytokinesis [20] (also seen at high concentrations of Y-27632 [10] ). We therefore evaluated the safety range of the concentrations of blebbistatin that does not affect cytokinesis of hPS cells. H9 hES cells were treated with blebbistatin at different concentrations (1.25–30 μM) in mTeSR and grown for 5 days. Cells were fixed and evaluated by immunocytochemistry using two antibodies, an antibody against β-actin to distinguish binucleated cells from cells undergoing normal cell division and an antibody against Oct3/4 to select undifferentiated cells. There were no abnormally binucleated cells at concentrations lower than 20 μM, whereas a minor fraction of the cells showed binucleation at 25 μM ( Fig. 5i ). At 30 μM, some colonies included multinucleated cells, although many of the cells still maintained a normal morphology ( Fig. 5i ). Nevertheless, it is important to maintain the concentrations of blebbistatin for hPS cell cultures at minimally sufficient levels to avoid any adverse effect. 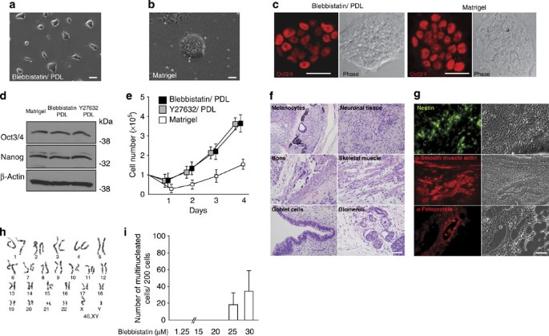Figure 5: Blebbistatin treatment supports self-renewal of hPS cells under a fully defined condition. (a–d) hiPS cells were grown on PDL in the presence of blebbistatin for 20 passages. Morphology of hiPS cells under blebbistatin/PDL condition (a) or standard feeder-free condition (Matrigel) (b) is shown. (c) Oct3/4 expression or phase contrast image of cells grown under blebbistatin/PDL conditions evaluated by immunofluorescence using confocal microscopy. (d) Oct3/4 and Nanog expression in cells grown under standard feeder-free (Matrigel), blebbistatin/PDL or Y-27632/PDL conditions was evaluated by immunoblot analysis. β-Actin was used as loading control. (e) The cell growth curve of hiPS cells cultured under blebbistatin/PDL, Y-27632/PDL or standard feeder-free (Matrigel) conditions was determined by counting the number of live cells. Each data point shows mean±s.d.,n=3. The population doubling time of cells grown under blebbistatin/PDL, Y-27632/PDL or standard feeder-free condition was approximately 32.1 h, 32.2 or 31.8 h, respectively. (f) Cells grown under blebbistatin/PDL condition for 20 passages were collected, and approximately 2×106cells were subcutaneously injected into SCID/beige mice. After 4–8 weeks, teratomas were collected and subjected to histological assessment. The presence of tissues derived from all three germ layers was confirmed in each teratoma sample. Scale bar, 100 μm. (g) The paraffin-embedded teratoma sections were examined by immunofluorescence analysis. Tissue-specific markers such as nestin, α-fetoprotein and α-smooth muscle actin were detected in teratoma-derived tissues. Scale bar, 100 μm. (h) hiPS(FS) cells grown under the defined condition (blebbistatin/PDL) for 20 passages were subjected to karyotyping by standard G-banding, and confirmed to maintain chromosomal integrity. (i) Binucleate cell analysis of hES cells treated with blebbistatin at different concentrations. H9 cells were grown on Matrigel-coated 12-well plates in mTeSR with 1.25–30 μM blebbistatin for 5 days. Cells were fixed and stained with β-actin and Oct3/4 antibodies. The number of multinucleated cells, which excludes cells undergoing normal cell division, was counted at each concentration. Data are mean±s.d.,n=3. Figure 5: Blebbistatin treatment supports self-renewal of hPS cells under a fully defined condition. ( a – d ) hiPS cells were grown on PDL in the presence of blebbistatin for 20 passages. Morphology of hiPS cells under blebbistatin/PDL condition ( a ) or standard feeder-free condition (Matrigel) ( b ) is shown. ( c ) Oct3/4 expression or phase contrast image of cells grown under blebbistatin/PDL conditions evaluated by immunofluorescence using confocal microscopy. ( d ) Oct3/4 and Nanog expression in cells grown under standard feeder-free (Matrigel), blebbistatin/PDL or Y-27632/PDL conditions was evaluated by immunoblot analysis. β-Actin was used as loading control. ( e ) The cell growth curve of hiPS cells cultured under blebbistatin/PDL, Y-27632/PDL or standard feeder-free (Matrigel) conditions was determined by counting the number of live cells. Each data point shows mean±s.d., n =3. The population doubling time of cells grown under blebbistatin/PDL, Y-27632/PDL or standard feeder-free condition was approximately 32.1 h, 32.2 or 31.8 h, respectively. ( f ) Cells grown under blebbistatin/PDL condition for 20 passages were collected, and approximately 2×10 6 cells were subcutaneously injected into SCID/beige mice. After 4–8 weeks, teratomas were collected and subjected to histological assessment. The presence of tissues derived from all three germ layers was confirmed in each teratoma sample. Scale bar, 100 μm. ( g ) The paraffin-embedded teratoma sections were examined by immunofluorescence analysis. Tissue-specific markers such as nestin, α-fetoprotein and α-smooth muscle actin were detected in teratoma-derived tissues. Scale bar, 100 μm. ( h ) hiPS(FS) cells grown under the defined condition (blebbistatin/PDL) for 20 passages were subjected to karyotyping by standard G-banding, and confirmed to maintain chromosomal integrity. ( i ) Binucleate cell analysis of hES cells treated with blebbistatin at different concentrations. H9 cells were grown on Matrigel-coated 12-well plates in mTeSR with 1.25–30 μM blebbistatin for 5 days. Cells were fixed and stained with β-actin and Oct3/4 antibodies. The number of multinucleated cells, which excludes cells undergoing normal cell division, was counted at each concentration. Data are mean±s.d., n =3. Full size image Although blebbistatin was originally discovered as a highly potent inhibitor for NMII (IC 50 =0.5–5 μM) without inhibiting class I, V and X myosin superfamily members [20] , it could affect other class II myosins of skeletal, cardiac and striated muscles in different species [35] . However, it is unlikely that these myosins have a major role in the cell death of hPS cells as they are not predominantly expressed in hES cells [27] ( Supplementary Table S2 ). Moreover, the data from stable knockdown of NMHCIIA in hES cells and NMHCIIA − /A − mES cells directly indicate the critical role of NMII in the regulation of cell death in pluripotent stem cells. The upstream regulator of NMII in cell death of hPS cells remains to be determined. Future studies will primarily focus on small GTPases such as RhoA [9] , [18] , [19] , which controls cellular interactions in hES cells [15] , and Cdc42, which is implicated in the regulation of nuclear movement [36] . It is also possible that in addition to NMII, ROCK may regulate cell death through interacting with other molecules. For instance, a recent study demonstrated that c-Jun N-terminal kinase, a known regulator of apoptosis, can be activated by ROCK in ultraviolet B-induced apoptosis [37] . Involvement of such a diverse set of cell death mechanisms may explain why the survival effect of blebbistatin or Y-27632 was variable depending on individual hPS cell lines. The use of blebbistatin could be advantageous in pinpointing NMII function over that of Y-27632, which is likely to affect numerous effector molecules downstream of ROCK [10] . In addition, blebbistatin is more cost-effective than Y-27632 for routine use. It has been suggested that fully reprogrammed hiPS cells can be generated in feeder-free conditions more efficiently than in traditional feeder-dependent culture conditions [38] . Thus, the novel culture method in our study may provide a basis to develop key technologies to efficiently derive and propagate new hiPS cell lines under fully defined conditions. Our data unexpectedly demonstrated that NMII seems to be connected to self-renewal programs in both human and mouse pluripotent stem cells mediated by unknown mechanisms. The early embryonic lethality of NMHCIIA − /A − mutant mice (E6.5) may be caused not only by impairment in cell adhesions but also by defects in differentiation programmes [24] . It is also plausible that NMII may function as a part of the molecular sensing machineries to monitor the surrounding niches that undergo drastic changes at physical and molecular levels during developmental processes. Understanding how multiple core functions of pluripotent stem cells are integrated by the motor protein NMII may shed light on the mechanistic link between cell architectural regulators and self-renewal networks, both of which constitute the basis of pluripotent stem cell identity. Furthermore, our results highlight NMII as a promising target to pharmacologically engineer the survival threshold of hPS cells. Chemicals Blebbistatin (±) (InSolution Blebbistatin), Blebbistatin (+), Blebbistatin (−), Y-27632 (InSolution Y-27632) and ML-7 were purchased from EMD. The compounds were always kept in the dark to avoid photoinactivation. When blebbistatin was used for cell culture, the exposure to fluorescent light for live-cell imaging was minimized to prevent phototoxicity. PDL was obtained from Millipore. Cell culture Two independent hES cell lines, H9 (WiCell) and BGN01 (BresaGen), were examined. A hES reporter line, BGN01v Oct4-GFP (Invitrogen), which stably expresses GFP under the Oct3 promoter, was also tested. hiPS cells used in the study include iPS(Foreskin) Clone 1 (WiCell) and two independently derived hiPS cells from normal human dermal fibroblasts, which have been characterized by a series of molecular and functional assays. For the regular feeder-free culture, hES or hiPS cells were grown on Matrigel (BD Biosciences)-coated plates in a defined medium, mTeSR (StemCell Technologies). For maintenance, cells were regularly passaged by the standard method using dispase (Invitrogen) or trypsin-EDTA (Lonza). BGN01v Oct4-GFP was maintained in the medium containing hygromycin (Invitrogen) at 10 μg ml −1 . For cell viability assay under the suspension condition, cells were grown in non-conditioned hES medium. hES medium (hESm) was prepared according to the following formula: DMEM/F12 (Invitrogen), 20% Knockout Serum Replacement (Invitrogen), 0.1 mM 2-mercaptoethanol (Sigma), 1 mM L -glutamine (Invitrogen), 4 ng ml −1 basic-FGF (Invitrogen) and 0.1 mM non-essential amino acids [31] , [39] . mES cells used in the experiment include CJ7, E14, RW4 (a parental line of NMHCIIA − /A − mES cells), NMHCIIA − /A − and NMHCIIB − /B − mES cells [24] , [26] . Cells were maintained on either mitotically inactivated mouse embryonic fibroblasts or gelatin (Sigma)-coated dishes with the standard medium in the presence of leukaemia inhibitory factor at 1,400 U ml −1 (Millipore) [40] . For the rescue experiment using NMHCIIA − /A − mES cells, cells were transiently transfected with GFP-tagged NMHCIIA plasmid using lipofectamine 2000 (Invitrogen), and subjected to immunoblot analysis and survival assay 2 days after transfection. For microscopic or immunofluorescence analysis, cells were plated at approximately 5,000–10,000 cells cm −2 . For the defined culture, cells were plated at approximately 10,000 cells cm −2 on plates freshly coated with PDL or PDL-precoated plates (BD Bioscience) in mTeSR supplemented with 2.5–5 μM of blebbistatin or Y-27632. The medium was changed every day or every other day depending on confluency. For passaging, cells were collected by using trypsin-EDTA, neutralized by trypsin neutralizing solution (Lonza) and pelleted by centrifugation, followed by one-time washing with Hank's balanced salt solution to completely remove residual trypsin. For the cell growth assay, hiPS or hES cells were plated at 2.5×10 4 cells cm −2 on plates coated with PDL or Matrigel in mTeSR in the presence of 5 μM blebbistatin or 5 μM Y-27632 (PDL) or in the absence of compounds (Matrigel). Cells were collected at the indicated time points, stained with Trypan blue and counted using a hemocytometer. Lentiviral vector-based shRNA knockdown in hES cells Lentiviral vector plasmids carrying a GFP reporter and shRNA sequences for human NMHCIIA were purchased from Open Biosystems. Lentiviral vectors were produced by transfecting the vector plasmids along with lentiviral packaging plasmids into 293T cells using lipofectamine 2000 (Invitrogen). After 24 h, the transfected cells were fed with fresh medium and grown for an additional 24 h. The culture supernatant containing the lentiviral vector was collected, filtered through a 0.45 μm filter syringe and added to BGN01 cells grown under feeder-free condition with 6 μg ml −1 polybrene. The fresh supernatant was also added to the cells on the following day. After 2–3 days, lentiviral vector infection was confirmed by GFP expression in cells using fluorescence microscopy. Cells were then treated with 1 μg ml −1 puromycin around 4 days after infection to selectively grow GFP-positive infected cells. GFP-positive colonies were manually picked up and further expanded in the presence of puromycin to establish individual knockdown lines. Each line was evaluated by immunoblot analysis to confirm efficient knockdown of NMHCIIA. Clonal assay hES or hiPS cells in mTeSR supplemented with or without blebbistatin were plated on Matrigel-coated 96-well plates at a single cell per well. Seven days after plating, cells were subjected to ALP assay using an Alkaline Phosphatase Detection Kit (Millipore) according to the manufacturer's instructions. The same cells were also evaluated by immunocytochemistry using an antibody against Oct3 (BD Bioscience). Cell viability assay hES or hiPS cells were collected by trypsinization, triturated by rigorous pipetting to obtain single cells and plated at 1×10 5 cells per well on 12-well plates coated with PDL or Matrigel in mTeSR in the presence or absence of blebbistatin or Y-27632 at various concentrations in triplicate. Dimethylsulphoxide (solvent for blebbistatin) was also added in the control condition and found to have no effect on viability. For mES cells, cells were plated under the same conditions, except for the use of gelatin coating and mES medium. After 24 h, cells were collected, trypsinized to single cells and counted using a hemocytometer. Cell counting was performed independently by two researchers to confirm the consistency. The same samples were used for TUNEL assay immediately after taking a small fraction of the sample for cell counting. For the evaluation of cell viability under suspension culture, hES or hiPS cells were trypsinized, rigorously triturated by extensive pipetting to obtain single cells and plated at 5×10 5 in non-tissue culture-treated six-well plates with non-conditioned standard hESm containing blebbistatin or Y-27632 at different concentrations in triplicate. After 24 or 48 h, cells were collected with trypsinization and extensive trituration by pipetting, and the number of live cells was manually counted using a hemocytometer and Trypan blue staining. The cell survival ratio (%) represents the ratio of the number of live cells to the number of cells plated. The same samples were subjected to TUNEL assay for side-by-side comparison with data from the cell viability assay. TUNEL assay The samples in triplicate used for cell viability assay were immediately tested by TUNEL assay using an APO-DIRECT kit (BD Pharmingen) according to the manufacturer's protocol. The number of TUNEL (FITC) or propidium iodide (PI)-positive cells was counted using a hemocytometer under fluorescence microscopy with a ×20 objective. When necessary, FITC-labelled cells were verified using a ×40 objective to exclude nonspecific signal. At least 300 cells were evaluated per sample and counting was repeated twice. The ratio of the number of TUNEL-positive cells to the number of PI-positive cells was calculated. The representative result was shown in the figure from experiments repeated at least three times. Although flow cytometric analysis was initially attempted, because of persistent cell aggregation in suspension culture even after extensive trypsinization and trituration, we decided to switch to manual cell counting, which correlated well with the data obtained from cell viability assay. Annexin-V binding assay BGN01vOct4-GFP cells were subjected to cell viability assay under the suspension condition in the presence or absence of 5 μM blebbistatin as described above. Cells were collected 24 h after plating, and incubated with annexin-V conjugated with Alexa-647 (BioLegend) at room temperature for 15 min according to the manufacturer's instructions, counterstained with PI and evaluated by fluorescence microscope. Approximately 150 cells per each condition in triplicate were examined to classify the cells into four categories, GFP (+)/annexin (+), GFP (+)/annexin (−), GFP (−)/annexin (+) and GFP (−)/annexin (−). Teratoma formation All animal-related protocols were approved by the Institutional Animal Care and Use Committee. Cells (approximately 2×10 6 cells) grown under defined conditions for multiple passages with occasional freezing and thawing were subcutaneously injected into SCID/beige mice (Charles River Laboratories). After 4–8 weeks, the developed teratomas were excised, fixed in 4% paraformaldehyde or 10% formalin and subjected to histological section preparations. Embryoid body formation Cells were obtained using dispase or trypsin-EDTA, plated on non-tissue culture treated dishes (approximately 10 6 cells per well per six-well plate) in the absence of compounds, and grown in non-conditioned hES medium for 14 days. Cells were collected for protein extraction, and subjected to immunoblot. Karyotyping Standard G-banded karyotyping was carried out for each cell line approximately every 10–20 passages [41] . Binucleation analysis H9 cells were plated on Matrigel-coated 12-well plates at 5×10 4 cells per well with various concentrations of blebbistatin ranging from 1.25 to 30 μM. After 5 days, cells were fixed in 4% paraformaldehyde and subjected to immunocytochemical analysis with antibodies against β-actin (Sigma) at 1:500 dilution and Oct3 (BD Biosciences) at 1:100 dilution. 4,6-Diamidino-2-phenylindole was used to counterstain the nuclei. In some experiments, blebbistatin was removed from the culture medium after 5 days of incubation, and cells were further grown for another 3 days in the absence of blebbistatin. Approximately 200 cells per each condition in triplicate were examined using the fluorescence microscope. Cells undergoing cytokinesis, as indicated by the presence of actin staining at the centre of the cell, were excluded from counting. Statistical analysis Biological replicates (3–5 replicates per condition) were subjected to statistical analysis by using analysis of variance or the paired t -test. Statistical significance was shown as the probability value such as ** P <0.01. Data points are shown as mean±s.d.